Developmental gene expression provides clues to relationships between sponge and eumetazoan body plans Elucidation of macroevolutionary transitions between diverse animal body plans remains a major challenge in evolutionary biology. We address the sponge-eumetazoan transition by analyzing expression of a broad range of eumetazoan developmental regulatory genes in Sycon ciliatum (Calcispongiae) . Here we show that many members of surprisingly numerous Wnt and Tgf β gene families are expressed higher or uniquely in the adult apical end and the larval posterior end. Genes involved in formation of the eumetazoan endomesoderm, such as β -catenin , Brachyury and Gata , as well as germline markers Vasa and Pl10 , are expressed during formation and maintenance of choanoderm, the feeding epithelium of sponges. Similarity in developmental gene expression between sponges and eumetazoans, especially cnidarians, is consistent with Haeckel’s view that body plans of sponges and cnidarians are homologous. These results provide a framework for further studies aimed at deciphering ancestral developmental regulatory networks and their modifications during animal body plans evolution. Elucidation of macroevolutionary transitions between animal body plans remains to be a major challenge in evolutionary biology [1] , [2] , [3] , [4] , additionally complicated by disputable branching order of metazoan lineages [5] , [6] . Several lines of evidence (morphology, molecular phylogenies, fossil record) suggest that the first multicellular animals had poriferan-grade body plans with choanoflagellate-like cells (choanocytes) used for water movement, food capture and digestion, but lacked key metazoan cell types, for example, nerves and muscles [7] , [8] , [9] , [10] , [11] , [12] . Some analyses support basal position of the ctenophores, morphological complexity of which might be a result of independent evolution [6] , [13] . Conversely, Trichoplax adhaerens, composed of only four cell types, appears to be secondarily simplified, as divergence of the placozoan lineage likely occurred after the divergence of sponges [14] . Thus, among the three contentious ‘basal’ clades, sponges, which likely retained the organization of the earliest metazoans, can be expected to provide significant clues towards understanding the origin of the complex bilaterian body plans [4] . Morphological and phylogenetic evidence makes the cnidarian polyps an ideal proxy to the ‘prebilaterian eumetazoan’ body organization, and cnidarian model systems reveal evolutionary ancestry of bilaterian characters [15] , [16] . The polyps are overtly radially symmetrical with a (generally) blind gut (gastrodermis) and apical oral opening. Developmental gene expression studies indicate that the gastrodermis is homologous to the bilaterian endoderm and mesoderm, although differences in regulatory networks between them exist [17] , [18] , [19] . Expression and function of Wnt genes in the larval posterior and the adult oral end of cnidarians, as well as the posterior end of multiple bilaterians, demonstrate that the main body axis is patterned by the Wnt pathway in both lineages [20] , [21] , [22] , [23] , [24] . Analysis of the Wnt pathway components expression in the adult Pleurobrachia , demonstrating nested Wnt expression in the oral region, suggests that this feature might also be shared with ctenophores [25] . The second (dorsal-ventral) body axis in bilaterians is patterned by bone morphogenetic protein ligands of the Tgfβ superfamily, which are also asymmetrically expressed along the directive axis of anthozoan cnidarians [26] , [27] . While Haeckel [28] , [29] directly compared the adult sponge body plans with those of corals, this view does not receive much support currently. One reason for such a discrepancy might be that Haeckel’s prime interests were calcareous sponges, many of which have asconoid or syconoid organization, at least superficially similar to cnidarian polyps: a columnar body composed of two epithelial layers with the inner layer serving a feeding function, and a single major opening (osculum) at the apical end. In contrast, the majority of sponge species are demosponges, including Amphimedon queenslandica , which currently serves as sponge representative in genomic studies [7] . Demosponges are characterized by more complex (leuconoid) body plans, with choanocyte chambers interlinked by endopinacocyte-lined canals, multiple exhalant canals, and usually appear amorphous in adult form. However, juveniles of demosponges are radially symmetrical with a single osculum and differ from the calcisponge juveniles only by having multiple choanocyte chambers [30] . To circumvent the problem of seemingly incomparable bauplans of adult sponges and eumetazoans, it has been suggested that eumetazoans are derived from sponge larvae [31] . While sponges have an extremely diverse array of larval types, all of them are non-feeding [30] , so evolution of cnidarian-grade organization from sponge larvae would require development of a feeding strategy in addition to paedogenesis. In contrast, direct evolution of cnidarian-grade organization from asconoid-like organization appears more parsimonious. Developmental gene expression analyses are informative in comparisons of cnidarian and bilaterian body plans as they provide the first clue to deciphering gene regulatory networks governing development [19] , [32] . True homology of structures can be revealed by involvement of conserved gene regulatory networks (conceptualized as kernels [2] or character identification networks [33] ) in their determination. A lack of robust methodologies for functional studies currently precludes establishment of gene regulatory networks in sponges, and these data only now begin to be available for cnidarians. However, identification and expression analysis of the candidate genes should allow determining whether the components of the eumetazoan gene regulatory networks are co-expressed during formation and maintenance of the putatively homologous structures in sponges. While absence of such genes in the genome, or absence of their coexpression, would indicate lack of conservation of the regulation, any observed coexpression of several network components can be treated as support (albeit not a proof) of homology. Importantly, the developmental gene toolkit of sponges is surprisingly similar to the eumetazoan toolkit, although information on its expression remains limited [4] , [7] . As a model system for this study, we use the calcaronean sponge Sycon ciliatum, for which we have generated sequence resources and developed protocols for studying gene expression [34] . We report identification of potentially informative developmental regulatory genes and their expression throughout development and during maintenance of the adult body. We use these expression data to discuss the notion of body plan homology between sponges and cnidarians proposed by Heackel and based on functional morphology. Our results provide a framework for further studies aimed at deciphering ancestral developmental regulatory networks and their modifications that underlie animal body plans evolution. Re-examination of development of S. ciliatum We revisited development of S. ciliatum , which is representative for calcaronean sponges [30] , [34] , [35] , [36] , [37] , [38] , [39] , [40] , and studied its local reproductive cycle. The adult specimens are syconoid, with choanocyte-lined radial chambers surrounding an atrial cavity and a single osculum (exhalant opening) at the apical end ( Fig. 1a–c ). Embryogenesis occurs in the mesohyl, between the outer pinacocyte and the inner choanocyte epithelia ( Fig. 1d–j ). 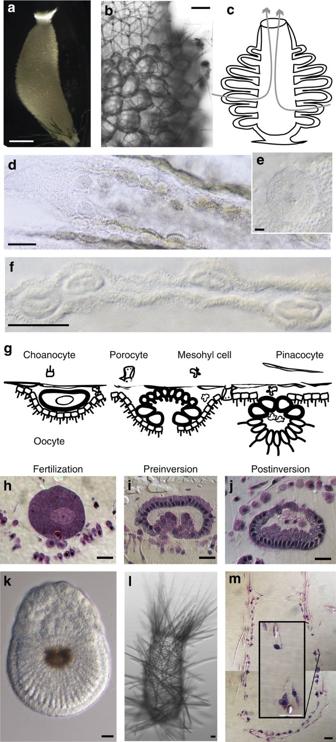Figure 1: Morphology and development ofSycon ciliatum. (a) Adult specimen attached to green algae with its basal part, osculum with fringe of spicules at the top. (b) Radial chambers of a juvenile specimen. (c) Syconoid body plan with direction of water flow indicated. (d,e) Fixed and cleared sample containing oocytes. (f) Fixed and cleared sample containing preinversion stage embryos. (g) Cartoon representation of major cell types and embryogenesis stages. (h–j) Histological sections demonstrating key embryogenesis stages. (k) Released live larva (macromeres on top, micromeres to the bottom). (l,m) Olynthus stage juvenile: live specimen and histological section demonstrating major cell types: choanocyte, pinacocyte and porocyte magnified in the inset. Scale bar indicates 5 mm ina, 100 μm inb,dandf, and 10 μm in remaining panels. Development is synchronous, and during the reproductive period ( Table 1 ) oocytes and embryos constitute a significant fraction of the sponge tissue ( Fig. 1d–f ). The larva ( Fig. 1k ) is composed of two major cell types: anterior ciliated micromeres and posterior non-ciliated macromeres. The larva also contains four cruciform cells distributed around its equator and a few cells of maternal origin inside of the larval cavity ( Fig. 1g,j ). During settlement, the anterior pole makes contact with the substrate; the micromeres differentiate into choanocytes and spicule producing cells; the macromeres differentiate into pinacocytes; the cruciform and maternal cells degenerate [36] . The osculum opens at the apical end and porocytes connecting choanoderm with pinacoderm differentiate, allowing water flow ( Fig. 1l,m ). At this stage (olynthus), the asconoid juvenile is the simplest filter-feeding multicellular animal. Radial chambers bud in a grossly radially symmetrical manner around the original choanocyte chamber, which becomes an endopinacocyte-lined atrial chamber ( Fig. 1b,c ). The radial chambers were suggested to correspond to complete olynthus-grade bodies attached with exhalant openings to the atrium, so that the apical-basal axis of polarity of the juvenile is reflected in proximal-distal axes of the radial chambers [40] . Figure 1: Morphology and development of Sycon ciliatum . ( a ) Adult specimen attached to green algae with its basal part, osculum with fringe of spicules at the top. ( b ) Radial chambers of a juvenile specimen. ( c ) Syconoid body plan with direction of water flow indicated. ( d , e ) Fixed and cleared sample containing oocytes. ( f ) Fixed and cleared sample containing preinversion stage embryos. ( g ) Cartoon representation of major cell types and embryogenesis stages. ( h – j ) Histological sections demonstrating key embryogenesis stages. ( k ) Released live larva (macromeres on top, micromeres to the bottom). ( l , m ) Olynthus stage juvenile: live specimen and histological section demonstrating major cell types: choanocyte, pinacocyte and porocyte magnified in the inset. Scale bar indicates 5 mm in a , 100 μm in b , d and f , and 10 μm in remaining panels. Full size image Table 1 Details of samples used for transcriptome assembly and quantification of expression. Full size table S. ciliatum homologues of eumetazoan developmental regulators We have searched the S. ciliatum genome and transcriptome sequences for potentially informative developmental regulatory genes, focusing on genes expressed during formation of the endomesoderm in cnidarians [19] , and Wnt and Tgfβ pathway components, involved in axial patterning in cnidarians and bilaterians [1] , [20] , [21] , [22] , [23] , [24] , [26] , [27] . Many genes involved in body plan patterning in cnidarians and bilaterians are conspicuously absent in Sycon (as they are in Amphimedon ): Twist , Snail , FoxA , FoxB , Otx , Dux , Blimp1 , Evx , Strabismus , Bicaudal , ElkA , Gsc , Six3/6 , FGFs and Sprouty . However, we have recovered 21 Wnt genes, multiple downstream components of the Wnt pathway, 22 Tgf β ligands, 6 Smad genes, two each of Vasa and Pl10 genes, and single Nanos , Gata , Gli and Hedgling genes. Sycon Tbox genes, including two Brachyurys , have been reported [41] . The surprisingly large number of Wnt genes stands in contrast to the situation in A. queenslandica , where only three Wnt genes are present [42] . We have also recovered eight Wnt sequences from the transcriptome of a homoscleromorph sponge, Oscarella sp [43] , two of them orthologous to previously published Oscarella lobularis genes [44] . While our analysis confidently places bilaterian and cnidarian Wnts into previously described subfamilies, sponge sequences (with exception of Amphimedon WntB and WntC loosely affiliated with Wnt8 subfamily) fall outside of the recognized eumetazoan subfamilies. We name the Sycon Wnts with consecutive letters ( WntA to WntU ) based on the order in which they were identified. Nine of the Sycon Wnt s form a well-supported clade affiliated with a single Oscarella sequence; smaller clades encompassing either Sycon or Oscarella genes are also recovered ( Supplementary Fig. 1 , Fig. 2a ), suggesting lineage-specific expansion events and obscuring the number of Wnt ligands in the last common ancestor. 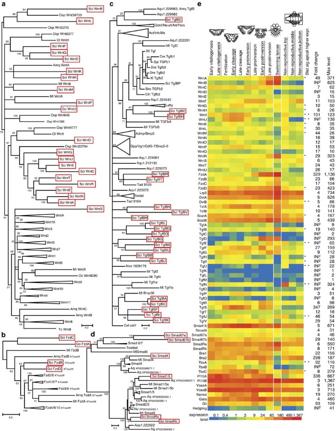Figure 2: Phylogenetic and expression analyses ofSycon ciliatumhomologues of genes involved in eumetazoan body plan patterning. Bayesian phylogenetic trees of selected identified genes (a–d) and heatmap showing expression profiles of all identified genes (e). (a–d) Sub-trees not containing sponge sequences are collapsed. Species: Ag,Anopheles gambiae, mosquito; Amq,Amphimedon queenslandica, demosponge; Av,Axinella verrucosa, demosponge; Bf,Branchiostoma floridae, cephalochordate; Ci,Ciona intestinalis, urochordate; Co,Capsaspora owczarzaki, unicellular opisthokont; Ct,Capitella teleta, polychete worm; Dm,Drosophila melanogaster, insect; Ef,Ephydatia fluviatilis, demosponge; Hm,Hydra magnipapillata, hydrozoan cnidarian; Hr,Helobdella robusta, leech; Lv,Lytechinus variegatus, echinoderm; Ml,Mnemiopsis leidyi, ctenophore; Mm,Mus musculus, vertebrate; Nv,Nematostella vectensis, anthozoan cnidarian; Ol,Oscarella lobularis, homoscleromorph sponge; Osp,Oscarellaspecies, homoscleromorph sponge; Om,Oopsacas minuta, hexactinellid sponge; Pc,Podocoryne carnea, hydrozoan cnidarian; Sci,Sycon ciliatum, calcareous sponge; Sd,Suberites domuncula, demosponge; Sm,Schmidtea mediterranea,planarian; Sp,Strongylocentrotus purpuratus, echinoderm; Sra,Sycon raphanus, calcareous sponge; Ta,Trichoplax adhaerens, placozoan; Tc,Tribolium castaneum, insect. The values at the tree nodes are posterior probabilities for each split defined over the range (0, 100). (e) Heatmap representation of expression profiles of the candidate genes calculated as sums of the posterior probability of each read coming from a given gene over all reads; early vitellogenesis to late postinversion samples are mid-body slices and contain both somatic tissue and reproductive elements/embryos; swimming larvae are released larvae without the maternal tissue; top, middle and bottom fragments were from sponges not containing reproductive elements; names of illustrated stages are underlined. The indicated fold changes and maximum level of expression relate to the entire expression profile. Statistically significant higher expression in the apical (top) region of the non-reproductive sponges in comparison to the middle or basal part is indicated by asterisks (left in comparison to the middle, right in comparison to the base). Figure 2: Phylogenetic and expression analyses of Sycon ciliatum homologues of genes involved in eumetazoan body plan patterning. Bayesian phylogenetic trees of selected identified genes ( a – d ) and heatmap showing expression profiles of all identified genes ( e ). ( a – d ) Sub-trees not containing sponge sequences are collapsed. Species: Ag, Anopheles gambiae , mosquito; Amq, Amphimedon queenslandica , demosponge; Av, Axinella verrucosa , demosponge; Bf, Branchiostoma floridae , cephalochordate; Ci, Ciona intestinalis , urochordate; Co, Capsaspora owczarzaki , unicellular opisthokont; Ct, Capitella teleta , polychete worm; Dm, Drosophila melanogaster , insect; Ef, Ephydatia fluviatilis , demosponge; Hm, Hydra magnipapillata , hydrozoan cnidarian; Hr, Helobdella robusta , leech; Lv, Lytechinus variegatus , echinoderm; Ml, Mnemiopsis leidyi , ctenophore; Mm, Mus musculus , vertebrate; Nv, Nematostella vectensis , anthozoan cnidarian; Ol, Oscarella lobularis , homoscleromorph sponge; Osp, Oscarella species, homoscleromorph sponge; Om, Oopsacas minuta , hexactinellid sponge; Pc, Podocoryne carnea , hydrozoan cnidarian; Sci, Sycon ciliatum , calcareous sponge; Sd, Suberites domuncula , demosponge; Sm, Schmidtea mediterranea, planarian; Sp, Strongylocentrotus purpuratus , echinoderm; Sra, Sycon raphanus , calcareous sponge; Ta, Trichoplax adhaerens , placozoan; Tc, Tribolium castaneum , insect. The values at the tree nodes are posterior probabilities for each split defined over the range (0, 100). ( e ) Heatmap representation of expression profiles of the candidate genes calculated as sums of the posterior probability of each read coming from a given gene over all reads; early vitellogenesis to late postinversion samples are mid-body slices and contain both somatic tissue and reproductive elements/embryos; swimming larvae are released larvae without the maternal tissue; top, middle and bottom fragments were from sponges not containing reproductive elements; names of illustrated stages are underlined. The indicated fold changes and maximum level of expression relate to the entire expression profile. Statistically significant higher expression in the apical (top) region of the non-reproductive sponges in comparison to the middle or basal part is indicated by asterisks (left in comparison to the middle, right in comparison to the base). Full size image All core components of the canonical Wnt pathway, except Axin , have been identified in Sycon : four Frizzled ( Fzd ) receptors, one Lrp5/6 co-receptor and two each of Dishevelled ( Dvl ), Tcf and β -catenins . Only two Fzds contain the KTxxxW motif, playing a role in transduction of the canonical signalling [45] , and these two ( FzdB and FzdD ) appear closely related to the eumetazoan and Amphimedon Fzds that also contain this motif. The only other known metazoan Fzd without this motif is the ctenophore Mnemiopsis FzdB [46] ( Supplementary Fig. 2 ; Fig. 2b ). We have carried out phylogenetic analysis of the 22 Sycon Tgf β superfamily ligands, adding these along with eight predicted Amphimedon protein sequences [7] to the dataset of Pang et al. [47] ( Supplementary Fig. 3 ; Fig. 2c ). The Sycon Tgf β repertoire includes one derived protein (TgfβD) containing the signalling C-terminal domain and a putative signal peptide, but no pre-protein domain. This sequence appears orthologous to pair of Amphimedon sequences, including the previously reported Tgf β [48] . SciTgf β P falls within the Tgf β sensu stricto subfamily together with two Amphimedon sequences and one ctenophore sequence. SciTgf β E and SciTgf β H , along with two ctenophore sequences, are weakly affiliated with Lefty genes. SciTgf β R and SciTgf β T cluster with one Amphimedon and one Trichoplax predicted proteins. The remaining sponge sequences fall out of the defined eumetazoan families ( Fig. 2c ). Two Sycon Smads are affiliated with the inhibitory Smads6/7 , one with co-Smad4 (a co-factor for receptor-specific Smads), one with Smads1/5 , and two are included within the receptor Smads group, but do not fall clearly into Smad2/3 or Smad1/5 family ( Supplementary Fig. 4 ; Fig. 2d ). In contrast, Amphimedon does not possess any Smads of the Smad6/7 subfamily. The single identified SciGata sequence clusters with AmqGata , and the two sequences fall between Gata1/2/3 and Gata4/5/6 subfamilies, indicating that the diversification of GATA family occurred after divergence of sponges ( Supplementary Fig. 5 and Supplementary Fig. 6 ). RNA-seq analysis of S. ciliatum gene expression We studied expression of the identified genes throughout the life cycle and across the main body axis of S. ciliatum using RNA-seq technology. We have taken advantage of the fact that embryonic development is semi-synchronous within a population, synchronous within individuals, and that oocytes and embryos occupy a significant fraction of the volume of the reproductive individuals ( Fig. 1d,f ; Table 1 ; Methods). Levels of gene expression were calculated as sums of the posterior probability of each read coming from a given gene over all reads, and the similarities and differences between samples calculated using available packages [49] , [50] . These analyses indicated expected similarities within replicates and distinctiveness of the samples isolated at different stages (except indistinguishable cleavage samples; Supplementary Figs 7 and 8 ). To visualize expression of the 73 identified genes during development and across the adult body axis, we generated a heatmap representation of expression ( Fig. 2e and Supplementary Fig. 9 ). Multiple genes including WntA , WntB, WntR, FzdA , Tgf β D and Hedgling are strongly upregulated in late embryogenesis and highly expressed in the larvae, while WntI , WntJ , TcfA , Tgf β S and Nanos have highest expression during cleavage. Almost all of the analyzed genes are expressed in somatic cells, as demonstrated by the presence of transcripts in samples derived from non-reproductive specimens, although expression of some genes (for example, WntB , Tgf β D , Hedgling and TboxB ) appears negligible in adult tissue as compared with developmental samples. We were particularly interested whether expression of Wnt and TGF β genes is associated with the apical-most (top) part of the sponge (osculum). We have thus calculated the statistical significance of the candidate genes’ expression being different in the apical part of the sponge, as described in [50] ( Supplementary Table 1 , Fig. 2e and Supplementary Fig. 9 ). Strikingly, among 21 Wnt genes and 22 TGF β genes, only one ( WntF ) was expressed significantly lower in the apical than the basal part, while nine Wnt genes and seven Tgf β genes were expressed significantly higher in the apical than the middle part. Expression of some of these genes was higher in the base of the sponge than in the middle, so that the apical expression was higher than basal, but without statistical significance. Thus, expression of two Wnt genes ( WntI , and WntJ ) and four Tgf β genes ( Tgf β E , Tgf β J , Tgf β N , Tgf β U ) was significantly higher in the apical part than in the middle and basal parts. Low expression of some ‘apical markers’ in the basal part of the sponge is not totally unexpected, as this region contains stolons providing attachment to the substrate and sometimes small secondary specimens (although none were present in the samples used for this study). In contrast, under normal conditions, additional axes are not generated along the body column. We thus consider comparisons between the top and middle region more informative. In contrast to ligands of the Wnt and TGFβ pathways, downstream components of these pathways, as well as other genes potentially involved in specification or maintenance of the choanoderm, were expressed more uniformly along the axis, with exceptions of β catA (higher in the top than in the middle) and DvlB (highest in the top). The Tbox family displayed highest diversity of expression profiles, with TboxA highest in the top, TboxC higher in the top than in the middle and Bra2 lowest in the top. Expression of Wnt pathway components in S. ciliatum The majority of Wnt genes are expressed in oocytes and uniformly in blastomeres during cleavage, but none was detected in preinversion stage embryos (for example, Fig. 3a–f ). WntF and WntB are strongly expressed in the maternal cells ingressing into the larval cavity ( Fig. 3g,h ). This expression of WntB persists in the compacted maternal cells positioned between the macromeres of the mature larvae ( Fig. 3h–j ). While maternal cell ingression superficially resembles gastrulation, these cells are not of embryonic origin and will degenerate before the juvenile sponge is formed [36] . WntA , WntB and WntR are expressed in the posterior half of the larvae: WntB in the macromeres, WntR in posterior most micromeres and WntA in macromeres and posterior most micromeres ( Fig. 3j–l ). WntJ , WntG , WntR and WntC are expressed in staggered domains around the osculum of adult sponges: WntJ in the apical-most outer epithelial cells of the oscular sphincter; WntG in a narrower ring of cells surrounding the WntJ domain; WntR in a ring of mesohyl cells around the osculum (and in rare mesohyl cells throughout the body column); and WntC in the ring of choanocytes on the border between the radial chambers and the region that remains in an asconoid organization, where formation of choanocyte chambers takes place ( Fig. 3m–t ). WntC is also expressed in the endopinacocytes of the atrial cavity, and, together with WntF , in cells surrounding the entries to the radial chambers ( Fig. 3u–v ), consistent with the notion that proximal-distal axes of chambers are homologous to the main body axis. WntM could be detected in a domain similar to WntG in only some specimens, likely because of its low-expression level. WntI is expressed in a variety of somatic cell types ( Fig. 3s ), and strongly in the embryos ( Fig. 3d ). We have not detected specific Wnt expression in exopinacoderm as reported for O. lobularis [44] , but low level expression of several Wnts does not exclude the possibility of such expression. Overall, the most prominent Wnt expression is associated with the posterior larval pole and apical/oscular poles of each of the modules constituting the body of Sycon : the osculum in the main body axis and the proximal ends of the radial chambers, and encompasses all three layers of the Sycon body (the outer pinacocyte layer: WntJ and WntG , the middle mesohyl layer: WntR , the inner choanocyte layer: WntC ). These patterns are strikingly reminiscent of the cnidarian larval posterior and adult oral Wnt expression domains. 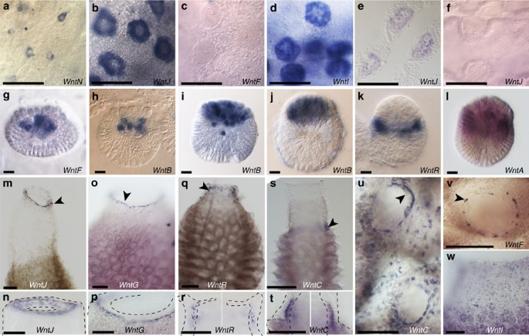Figure 3:In situhybridization detection of selectedWntgenes expression inSycon ciliatum. (a) Expression ofWntNin small oocytes. (b) Expression ofWntJin large oocytes. (c) Large oocytes negative forWntFexpression. (d,e) uniform expression ofWntIandWntJduring cleavage. (f) Expression ofWntJis undetectable in preinversion embryos. (g,h)WntFandWntBare expressed in maternal cells inside of postinversion embryos. (i,j) Maternal cells become compact and squeezed between macromeres during maturation of the larvae, while the macromeres start to expressWntB;iis a nearly-mature larva isolated from the parent sponge,jis a free-swimming larva. (k) A narrow band of posterior most micromeres expressesWntR. (l) Macromeres and posterior most micromeres expressWntA. (m,n)WntJis specifically expressed in the very tip of the osculum, including the oscular sphincter. (o,p)WntGis expressed in cells surroundingWntJexpression domain. (q,r)WntRis expressed in a band of mesohyl cells just under the sphincter. (s,t)WntCis expressed in a stripe encompassing forming choanocyte chambers. (u,v) View of endopinacoderm lining the atrial cavity and entry to the radial chambers:WntCis broadly expressed in this region, whileWntFis expressed only in the cells directly lining the entrance to the radial chambers. (w) WntI is broadly expressed in a variety of cell types. Embryos and larvae in panelsg–lare positioned with anterior pole towards the bottom. Scale bar represents 100 μm except panelsg–l, where it represents 10 μm. Figure 3: In situ hybridization detection of selected Wnt genes expression in Sycon ciliatum . ( a ) Expression of WntN in small oocytes. ( b ) Expression of WntJ in large oocytes. ( c ) Large oocytes negative for WntF expression. ( d , e ) uniform expression of WntI and WntJ during cleavage. ( f ) Expression of WntJ is undetectable in preinversion embryos. ( g , h ) WntF and WntB are expressed in maternal cells inside of postinversion embryos. ( i , j ) Maternal cells become compact and squeezed between macromeres during maturation of the larvae, while the macromeres start to express WntB ; i is a nearly-mature larva isolated from the parent sponge, j is a free-swimming larva. ( k ) A narrow band of posterior most micromeres expresses WntR . ( l ) Macromeres and posterior most micromeres express WntA . ( m , n ) WntJ is specifically expressed in the very tip of the osculum, including the oscular sphincter. ( o , p ) WntG is expressed in cells surrounding WntJ expression domain. ( q , r ) WntR is expressed in a band of mesohyl cells just under the sphincter. ( s , t ) WntC is expressed in a stripe encompassing forming choanocyte chambers. ( u , v ) View of endopinacoderm lining the atrial cavity and entry to the radial chambers: WntC is broadly expressed in this region, while WntF is expressed only in the cells directly lining the entrance to the radial chambers. ( w ) WntI is broadly expressed in a variety of cell types. Embryos and larvae in panels g – l are positioned with anterior pole towards the bottom. Scale bar represents 100 μm except panels g – l , where it represents 10 μm. Full size image While the posterior-anterior gradient of expression of Wnt ligands in larval and adult eumetazoans reflects the conserved role in axial patterning, the earliest function of the canonical Wnt pathway (signalling through β-catenin) is specification of the endomesoderm [19] , [51] , [52] . We thus studied expression of downstream components of the pathway ( Figs 4 and 5 ). FzdB, FzdC and FzdD are expressed uniformly in the oocytes and cleavage stage embryos, while FzdA and FzdD in the embryonic and larval micromeres ( Fig. 4a–p ). FzdC and FzdD are expressed in choanocytes and a fraction of mesohyl cells, and FzdD additionally in a ring of mesohyl cells surrounding the osculum ( Fig. 4m,q ). Both Dvl homologues are expressed strongly in the oocytes; their expression decreases during cleavage in most cells, remaining high in the cruciform cells ( Fig. 4r,s,v,w ). DvlA is expressed in micromeres, choanocytes, and a fraction of mesohyl cells, including prominent ring surrounding the osculum ( Fig. 4t–u ). DvlB is expressed strongest in the region where choanocyte chambers are forming ( Fig. 4y ). Lrp5/6 is expressed in choanocytes, small oocytes and embryos, with exception of cleavage stages ( Fig. 5a–d ). Both Tcf genes are expressed throughout the choanocytes, upregulated in oocytes and ubiquitously expressed in the embryos, with TcfB stronger in the cruciform cells ( Fig. 5e–l ). 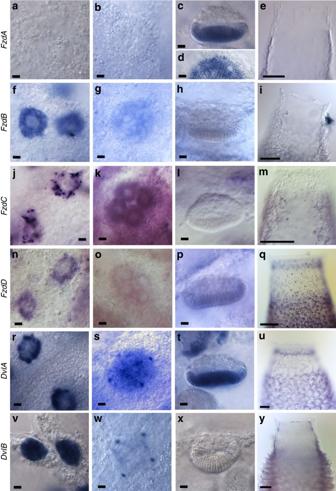Figure 4:In situhybridization detection ofFzdandDvlgenes inSycon ciliatum. Columns from left to right show: oocytes, cleavage, postinversion (side view with anterior pole towards bottom exceptd, which is a top view) and top (osculum) region of adult sponges. (a–e)FzdAis expressed uniquely in embryonic micromeres. (f–i)FzdBis expressed in oocyte and in cleavage stage embryos. (j–m)FzdCis expressed in oocyes, cleavage stage embryos, choanocytes and a fraction of mesohyl cells. (n–q)FzdDis expressed uniformly throughout early development before becoming restricted to micromeres; in adult sponges transcripts are localized to choanocytes and a range of mesohyl cells including prominent ring under the osculum. (r–u)DvlAis expressed in oocytes and cleavage stage embryos with stronger expression in cruciform cells, then becomes restricted to micromeres in postinversion stage embryos; in adult sponges prominent ring under the osculum as well as radial chambers expression are apparent. (v–y) Early expression ofDvlBis similar toDvlA, but no expression is detectable in older embryos, and in adults expression is most prominent in the uppermost radial chambers. Scale bars represent 10 μm except the right column, where they represent 100 μm. Figure 4: In situ hybridization detection of Fzd and Dvl genes in Sycon ciliatum . Columns from left to right show: oocytes, cleavage, postinversion (side view with anterior pole towards bottom except d , which is a top view) and top (osculum) region of adult sponges. ( a – e ) FzdA is expressed uniquely in embryonic micromeres. ( f – i ) FzdB is expressed in oocyte and in cleavage stage embryos. ( j – m ) FzdC is expressed in oocyes, cleavage stage embryos, choanocytes and a fraction of mesohyl cells. ( n – q ) FzdD is expressed uniformly throughout early development before becoming restricted to micromeres; in adult sponges transcripts are localized to choanocytes and a range of mesohyl cells including prominent ring under the osculum. ( r – u ) DvlA is expressed in oocytes and cleavage stage embryos with stronger expression in cruciform cells, then becomes restricted to micromeres in postinversion stage embryos; in adult sponges prominent ring under the osculum as well as radial chambers expression are apparent. ( v – y ) Early expression of DvlB is similar to DvlA , but no expression is detectable in older embryos, and in adults expression is most prominent in the uppermost radial chambers. Scale bars represent 10 μm except the right column, where they represent 100 μm. 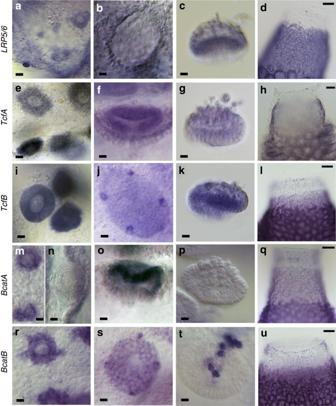Figure 5:In situhybridization detection of the canonical Wnt pathway components inSycon ciliatum. Columns from left to right show: oocytes, cleavage (top view,b,j,s) or preinversion (side view,fando), postinversion (side view with anterior pole towards bottom) and top (osculum) region of adult sponges. (a–d),Lrp5/6is expressed in small and medium sized oocytes, throughout postinversion stage embryos and in choanocytes. (e–l) BothTcfgenes are expressed throughout the development and in choanocytes, withTcfBbeing particularly prominent in the cruciform cellsj. (m–q)BcatAis expressed in medium sized but not mature oocytes, in micromeres before but not after inversion, and in choanocytes and range of mesohyle cells. (r–u)BcatBis expressed in oocytes and during cleavage with stronger expression in cruciform cells, then in the maternal cells ingressing into larval cavity, and in choanocytes and range of mesohyle cells. Scale bars represent 10 μm except the right column, where they represent 100 μm. Full size image Figure 5: In situ hybridization detection of the canonical Wnt pathway components in Sycon ciliatum . Columns from left to right show: oocytes, cleavage (top view, b , j , s ) or preinversion (side view, f and o ), postinversion (side view with anterior pole towards bottom) and top (osculum) region of adult sponges. ( a – d ), Lrp5/6 is expressed in small and medium sized oocytes, throughout postinversion stage embryos and in choanocytes. ( e – l ) Both Tcf genes are expressed throughout the development and in choanocytes, with TcfB being particularly prominent in the cruciform cells j . ( m – q ) BcatA is expressed in medium sized but not mature oocytes, in micromeres before but not after inversion, and in choanocytes and range of mesohyle cells. ( r – u ) BcatB is expressed in oocytes and during cleavage with stronger expression in cruciform cells, then in the maternal cells ingressing into larval cavity, and in choanocytes and range of mesohyle cells. Scale bars represent 10 μm except the right column, where they represent 100 μm. Full size image Both β -catenin genes are dynamically expressed: β catA in young oocytes, but not in mature oocytes undergoing fertilization nor during cleavage, upregulated in the micromeres of preinversion stage embryos and decreasing after inversion ( Fig. 5m–p ); β catB in oocytes of all sizes and in early embryos (higher in the cruciform cells) and then in the maternal cells ( Fig. 5r–t ). Both β -catenins are expressed in choanocytes and a ring of mesohyl cells surrounding the osculum ( Fig. 5q,u ). Thus, all key components of the canonical Wnt pathway are expressed in the choanoderm+mesohyl lineage, including the embryonic and larval micromeres as well as mature choanocytes and mesohyl cells. Expression of Tgfβ pathway components in S. ciliatum Several Tgf β ligands are expressed uniformly in oocytes and cleavage stage embryos (for example, Fig. 6a–d ). Tgf β D is strongly and specifically expressed in the embryonic and larval macromeres ( Fig. 6e,f ). In postinversion stage embryos, Tgf β F is expressed in the macromeres, and, along with Tgf β G and Tgf β B, is detectable in the maternal cells ( Fig. 6g–i ). In adults, expression of Tgf β B is uniform in the choanocytes and high in a few cells within the oscular sphincter ( Fig. 6j–k ). The most prominent region of Tgf β expression is the top/apical region, with strong expression of Tgf β N (also expressed in the entries of the radial chambers), Tgf β H , Tgf β E , Tgf β U and Tgf β J detected in a variety of cell types around the osculum ( Fig. 6l–q ). Thus, expression of Tgf β superfamily ligands is similar to expression of Wnt ligands in Sycon: predominantly posterior in the larvae and apical in the adults. 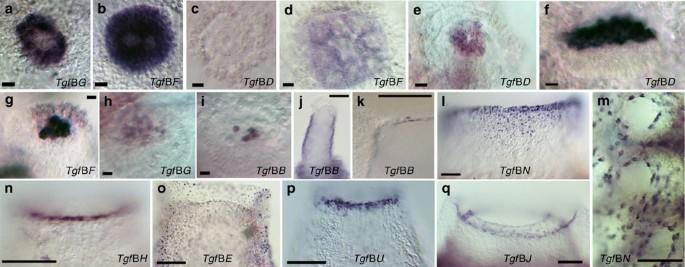Figure 6:In situhybridization detection ofTgfβ ligands inSycon ciliatum. (a–c) Oocytes (positive forTgfβGandTgfβF, but notTgfβD). (d) 8-cell stage embryo positive forTgfβF. (e,f) Macromeres positive forTgfβDin pre and postinversion stage embryos. (g–i) Postinversion stage embryos demonstrating maternal cells positive forTgfβF(also expressed in the macromeres, top),TgfβGand TgfβB. (j) Top part of very young adult with choanocytes positive forTgfβB.(k) rareTgfβB-positive cells residing in the oscular sphincter. (l,m)TgfβNexpression around the osculum and at the bases of radial chambers. (n–q) Top parts of sponges displaying expression ofTgfβ ligands. Scale bars represent 10 μm ina–jand 100 μm inl–q. Figure 6: In situ hybridization detection of Tgf β ligands in Sycon ciliatum. ( a – c ) Oocytes (positive for Tgf β G and Tgf β F , but not Tgf β D ). ( d ) 8-cell stage embryo positive for Tgf β F . ( e , f ) Macromeres positive for Tgf β D in pre and postinversion stage embryos. ( g – i ) Postinversion stage embryos demonstrating maternal cells positive for Tgf β F (also expressed in the macromeres, top), Tgf β G and TgfβB. ( j ) Top part of very young adult with choanocytes positive for Tgf β B. ( k ) rare Tgf β B -positive cells residing in the oscular sphincter. ( l , m ) Tgf β N expression around the osculum and at the bases of radial chambers. ( n – q ) Top parts of sponges displaying expression of Tgf β ligands. Scale bars represent 10 μm in a – j and 100 μm in l – q . Full size image We have next studied expression of the key Sycon Smad genes: Smad1/5 and Smad4 , implicated in endomesoderm specification in the cnidarians [19] and one of the ‘basal receptor smads’, SmadRa . Among them, Smad1/5 displayed the most dynamic expression: strong in the oocytes, restricted to the cruciform cells and the macromeres of preinversion and early postinversion stage embryos, and confined to the micromeres of late postinversion stage embryos ( Fig. 7a–e ). In adults, low expression was detectable in the choanocytes ( Fig. 7f ). Expression of Smad4 was uniform in oocytes, throughout the cleavage and in preinversion stage embryos, then detectable only in the maternal cells of early postinversion stage embryos, and strong in the micromeres of later postinversion embryos ( Fig. 7g–k ). In the adults, lower expression of Smad4 could be detected in choanocytes and mesohyl cells ( Fig. 7l ). SmadRa was expressed weakly in the oocytes and throughout cleavage, and prominent in the maternal cells in postinversion stage embryos ( Fig. 7m–q ). In adults, the expression could be detected in choanocytes and mesohyl cells, particularly those around the osculum. Thus, Smad genes were expressed either in the same or cells adjacent to those expressing Tgf β ligands. 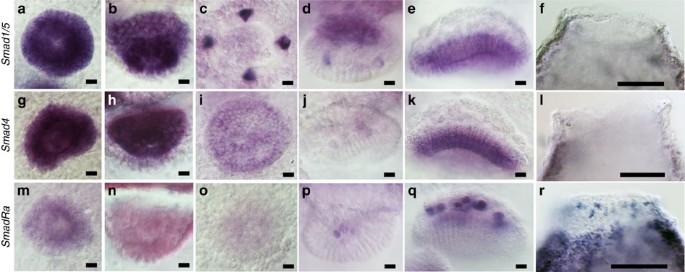Figure 7:In situhybridization detection of keySmadgenes inSycon ciliatum. Columns from left to right: large oocyte, late cleavage (side view), early preinversion (top view), early postinversion (side view), late postinversion (side view) and top parts of adult sponges. (a–f)Smad1/5is expressed dynamically throughout development with prominent expression in cross cells, early postinversion macromeres and late postinversion micromeres, and in choanocytes. (g–l)Smad4expression is similar toSmad1/5except less pronounced cross cells expression and presence of transcripts in maternal cells. (m–r)SmadRaexpression is predominant in maternal cells within embryos, mesohyl cells and choanocytes. Scale bars represent 10 μm exceptf,landr, where they represent 100 μm. Figure 7: In situ hybridization detection of key Smad genes in Sycon ciliatum . Columns from left to right: large oocyte, late cleavage (side view), early preinversion (top view), early postinversion (side view), late postinversion (side view) and top parts of adult sponges. ( a – f ) Smad1/5 is expressed dynamically throughout development with prominent expression in cross cells, early postinversion macromeres and late postinversion micromeres, and in choanocytes. ( g – l ) Smad4 expression is similar to Smad1/5 except less pronounced cross cells expression and presence of transcripts in maternal cells. ( m – r ) SmadRa expression is predominant in maternal cells within embryos, mesohyl cells and choanocytes. Scale bars represent 10 μm except f , l and r , where they represent 100 μm. Full size image Expression of Tbox genes in S. ciliatum The Tbox transcription factor Brachyury is essential for formation of endomesoderm, and in a variety of bilaterians and cnidarians is expressed in future endomesodermal cells as they move through the blastopore [17] . Expression of Wnts and Brachyury overlaps in the posterior region of cnidarian embryos where the blastopore is located, and persists in the cnidarian oral/apical end. Several other Tbox family genes, including the Eomes class, are also involved in formation of the endomesoderm [53] . We have recently reported the presence and eumetazoan-like properties of two Brachyury homologues, and the presence of Eomes and basal class Tboxes in Sycon [41] . Here we report expression of these genes. SciBra1 is expressed weakly in the oocytes and is undetectable in early preinversion stage embryos ( Fig. 8a ). In late preinversion stage embryos strong expression is apparent in the micromeres adjacent to the macromeres ( Fig. 8b–d ). Bra2 is expressed strongly in the oocytes, weaker during cleavage and slightly stronger in the micromeres than macromeres during preinversion ( Fig. 8f–i ). Both Brachyury genes are expressed uniformly in the choanocytes. One of Eomes -class Sycon Tboxes, TboxA , is not expressed embryonically, but instead marks accessory cells (derived from choanocytes) associated with pre and postinversion embryos ( Fig. 8k–n ). In the adults, its expression is localized only around the opening of the oscular sphincter ( Fig. 8o,p ). The second Eomes -class TboxB is expressed uniquely in the oocytes ( Fig. 8q ). TboxC, which belongs to the newly defined Tbox7 subfamily [32] , is expressed in the oocytes, throughout cleavage, and in preinversion stage embryos (stronger in the micromeres) ( Fig. 8r–u ). In adults, TboxC is expressed in a fraction of mesohyl cells, particularly at the tips of uppermost radial chambers ( Fig. 8v ). Thus, the predominant expression of Sycon Tbox genes is associated with micromeres as they translocate through the opening between macromeres and accessory cells, as well as choanocytes and mesohyl cells of the adult sponges. 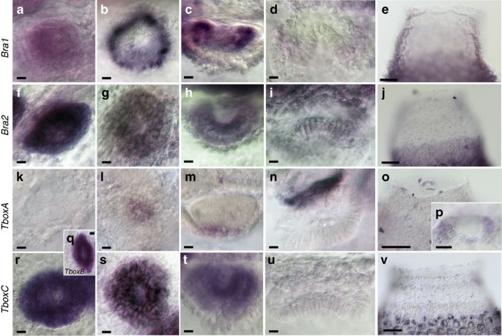Figure 8:In situhybridization detection ofTboxgenes inSycon ciliatum. Columns from left to right: large oocytes, top and side views of preinversion stage embryos, side view of early postinversion stage embryos, top parts of adults. (a–e)Bra1is most prominent in a ring of micromeres just before inversion; it is also weakly expressed in oocytes and choanocytes. (f–j)Bra2is expressed strongly in oocytes and younger embryos, and in choanocytes. (k–o)TboxAis expressed in accessory cells and around oscular opening. (q),TboxBis expressed in oocytes. (r–v)TboxCis expressed asBra2in oocytes and embryos, and then strongly in cells at tips of uppermost radial chambers. Scale bars represent 10 μm excepte,j,oandv, where they represent 100 μm. Figure 8: In situ hybridization detection of Tbox genes in Sycon ciliatum. Columns from left to right: large oocytes, top and side views of preinversion stage embryos, side view of early postinversion stage embryos, top parts of adults. ( a – e ) Bra1 is most prominent in a ring of micromeres just before inversion; it is also weakly expressed in oocytes and choanocytes. ( f – j ) Bra2 is expressed strongly in oocytes and younger embryos, and in choanocytes. ( k – o ) TboxA is expressed in accessory cells and around oscular opening. ( q ), TboxB is expressed in oocytes. ( r – v ) TboxC is expressed as Bra2 in oocytes and embryos, and then strongly in cells at tips of uppermost radial chambers. Scale bars represent 10 μm except e , j , o and v , where they represent 100 μm. Full size image Expression of additional endomesoderm specification genes In Nematostella embryos, the eumetazoan germline markers Vasa , Pl10 and Nanos2 are expressed in the presumptive endoderm and their expression responds to up or downregulation of the canonical Wnt pathway, consistent with a role in endomesoderm specification [19] , [54] . In contrast, NvNanos1 is expressed in nematocyst precursors, consistent with the neuronal expression of Nanos genes in other cnidarians and bilaterians [54] , [55] . As expected for germline markers, all of the identified Sycon homologues of Pl10 , Vasa and Nanos are expressed in oocytes ( Fig. 9a,e,i ). Expression of Pl10A decreases during cleavage ( Fig. 9b–d , top), but Pl10B expression remains strong and uniform in embryos, larvae and then choanocytes ( Fig. 9b–d , bottom). Both Vasa genes are expressed throughout the embryos, with expression elevated in the cruciform cells of preinversion stage embryos and micromeres of postinversion stage embryos ( Fig. 8f,g ). VasaB is also strongly expressed in the choanocytes ( Fig. 9h ). SciNanos is expressed in the macromeres and cross cells during preinversion ( Fig. 9j ) and is undetectable in the somatic cells of the adult sponges ( Fig. 9k–l ). 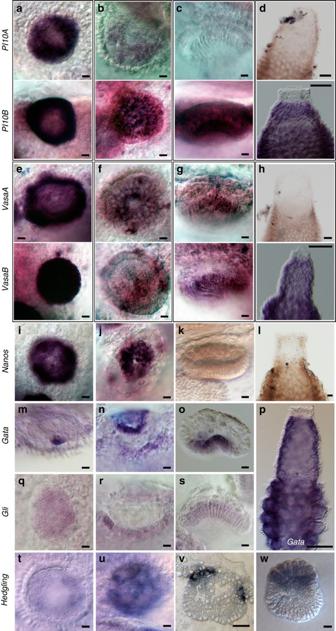Figure 9:In situhybridization detection ofSycon ciliatumhomologues of genes implicated in endomesoderm specification. Columns from left to right: large oocytes, cleavage to preinversion (top view exceptnandr, which are side views), postinversion (side view), top parts of young adult sponges (exceptw, larva). (a–d)Pl10Ais expressed uniquely in oocytes and early cleavage stage embryos, whilePl10Bthroughout development and in choanocytes. (e–h) BothVasagenes are expressed throughout development with prominent cross cells expression;VasaBis expressed in choanocytes. (i–l)Nanosis expressed in oocytes and then restricted to macromeres and cross cells of preinversion stage embryos. (m–p)Gatais expressed in the cells of fertilization complex, accessory cells, central/anterior micromeres and choanocytes. (q–s)Gliis expressed in oocytes, choanocytes and postinversion micromeres. (t–u)Hedglingis expressed in oocytes and during cleavage, and then in embryonic and larval macromeres. Scale bars represent 10 μm exceptd,h,landp, where they represent 100 μm. Figure 9: In situ hybridization detection of Sycon ciliatum homologues of genes implicated in endomesoderm specification. Columns from left to right: large oocytes, cleavage to preinversion (top view except n and r , which are side views), postinversion (side view), top parts of young adult sponges (except w , larva). ( a – d ) Pl10A is expressed uniquely in oocytes and early cleavage stage embryos, while Pl10B throughout development and in choanocytes. ( e – h ) Both Vasa genes are expressed throughout development with prominent cross cells expression; VasaB is expressed in choanocytes. ( i – l ) Nanos is expressed in oocytes and then restricted to macromeres and cross cells of preinversion stage embryos. ( m – p ) Gata is expressed in the cells of fertilization complex, accessory cells, central/anterior micromeres and choanocytes. ( q – s ) Gli is expressed in oocytes, choanocytes and postinversion micromeres. ( t – u ) Hedgling is expressed in oocytes and during cleavage, and then in embryonic and larval macromeres. Scale bars represent 10 μm except d , h , l and p , where they represent 100 μm. Full size image GATA transcription factors are regulators of endomesoderm development, although in Nematostella endodermal Gata expression starts after the endoderm is already formed, indicating that it is not part of the endomesoderm specification kernel in this cnidarian [18] , [19] . SciGata expression is undetectable in the oocytes ( Fig. 9m ), but is strong in the central/anterior micromeres ( Fig. 9n–o ). In adults, Gata is expressed in choanocytes ( Fig. 9p ), and is additionally upregulated in choanocyte-derived cells of the fertilization complex and the accessory cells ( Fig. 9m–n ). Hedgehog signalling is involved in endomesoderm formation in bilaterians, and the key transcription factor of the pathway, Gli , is expressed in the presumptive endoderm of Nematostella [19] , [56] . SciGli is expressed in the oocytes and micromeres of postinversion stage embryos ( Fig. 9q–s ). In adults, Gli is expressed in the choanocytes ( Fig. 9r ). We have not found a true Hedgehog gene in Sycon (none is present in Amphimedon [57] ), and it is yet to be known whether Hedgling signals through Gli . Nonetheless, we have studied expression of SciHedgling as the possible activator of Gli . SciHedgling is detectable from fertilization, becomes strong during cleavage, is then restricted to the macromeres and not detected in the somatic tissue ( Fig. 9t–v ). Thus, in Sycon embryos and larvae, but not in the adults, Hedgling is expressed in cells adjacent to those expressing Gli . Almost 150 years ago, Haeckel proposed that the body plans of sponges and corals are basically the same: the inner layer serves the digestive function and is the source of gametes, and the outer layer serves the protective and sensory functions [28] . Since then, no other hypothesis on the relationship of the adult body plans between sponges and the eumetazoans has been put forward, and the prevailing view appears to be that these body plans are incomparable. To test whether the body axes and the germ layers are homologous, we need to know whether conserved gene regulatory networks are involved in their determination. Expression analysis of the putative network components is the first step to identification of the interaction partners. In this study we performed a comprehensive expression analysis of calcisponge homologues of genes involved in axial patterning and endomesoderm formation in eumetazoans, especially cnidarians [1] , [18] , [19] , [20] , [32] . We hypothesized that sponge larval posterior and adult apical (peri-oscular) expression of genes expressed in (and constituting parts of networks involved in determination of) the posterior and oral end of the cnidarian polyps would be consistent with the homology of embryonic and adult axes, respectively. At the same time, expression of eumetazoan endomesodermal regulators in embryonic/larval sponge cells destined to differentiate into choanocytes, and in choanocytes of adults, would be consistent with homology of the germ layers between sponges and the eumetazoans. In bilaterians and cnidarians, expression of Wnt ligands is associated with and involved in patterning of the posterior and oral end [20] , [21] , [22] , [23] , [24] . Expression of Tgf β ligands, especially of the BMP family, marks the perpendicular axis in bilaterians and anthozoan cnidarians, while it is symmetrical around the hypostome of radial cnidarian polyps like Hydra [26] , [27] , [58] . One of the three Amphimedon Wnt ligands is specifically expressed in the posterior pole of the embryos and larvae, and one of the eight Amphimedon Tgf β ligands is expressed in the outer embryonic layer, and then restricted to the posterior pole [7] , [48] . Nothing is known about the expression of relevant genes in juvenile or adult demosponges, but transplantation experiments performed with Ephydatia mulleri demonstrated organizer properties of the osculum, and that this activity is likely conveyed by canonical Wnt signalling [59] . We have not been able to replicate this result in Sycon , possibly because Ephydatia, like the overwhelming majority of sponges, produces multiple oscula as it grows, while Sycon evolved mechanisms preserving a single body axis throughout its life. Our expression analysis demonstrates that as in Amphimedon , Wnt and Tgf β ligands are expressed in the posterior region of Sycon larvae ( Fig. 10a,b ). This expression is not limited to a specific cell type, as macromeres, posterior-most micromeres and maternal cells express these genes. These patterns are reminiscent of the nested expression domains of Wnt ligands in the Nematostella embryos [20] . Significantly, multiple Wnt and Tgf β ligands are expressed around the osculum of Sycon in a series of nested domains encompassing all three tissue layers. Moreover, Wnt and Tgf β ligands are expressed at the bases of radial chambers, which are serially homologous to the original juvenile body unit ( Fig. 10f ). Thus, larval and adult expression of Wnt and Tgf β ligands along the anterior-posterior and apical-basal axes is consistent with homology of the axes between sponges and cnidarian polyps. 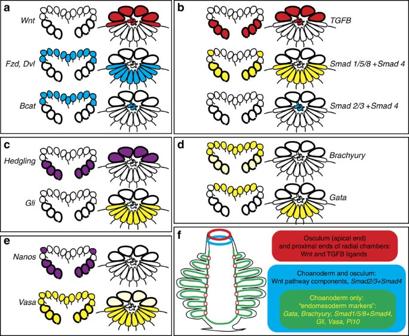Figure 10: Summary of embryonic and adult expression patterns obtained in this study. (a–e) Embryonic expression is depicted for preinversion and postinversion stage embryos, as in earlier stages expression was uniform if detected. (a) Wnt pathway; (b) TGFβ pathway; (c) putative hedgling pathway; (d) transcription factors implicated in endomesoderm specification in bilaterians; (e) germline markers implicated in endomesoderm specification in cnidarians; (f) combination of expression domains in adult sponges. In all panels,WntandTgfβ ligands expression is indicated in red, expression of canonical Wnt pathway components in blue, expression of remaining ‘endomesodermal markers’, which continue to be expressed in choanoderm is yellow. Green indicates coexpression of ‘blue’ and ‘yellow’ markers.HedglingandNanos(purple) can only be detected embryonically. Figure 10: Summary of embryonic and adult expression patterns obtained in this study. ( a – e ) Embryonic expression is depicted for preinversion and postinversion stage embryos, as in earlier stages expression was uniform if detected. ( a ) Wnt pathway; ( b ) TGFβ pathway; ( c ) putative hedgling pathway; ( d ) transcription factors implicated in endomesoderm specification in bilaterians; ( e ) germline markers implicated in endomesoderm specification in cnidarians; ( f ) combination of expression domains in adult sponges. In all panels, Wnt and Tgf β ligands expression is indicated in red, expression of canonical Wnt pathway components in blue, expression of remaining ‘endomesodermal markers’, which continue to be expressed in choanoderm is yellow. Green indicates coexpression of ‘blue’ and ‘yellow’ markers. Hedgling and Nanos (purple) can only be detected embryonically. Full size image While analyzing germ layer-specific expression in sponges, it is important to note that the presumptive choanoderm cells are located on the outside of the larvae and are used in larval locomotion. Thus, the formation of the choanoderm (which would equal gastrulation if choanoderm was homologous to the endomesoderm) is a multi-step process. First, the presumptive choanoderm cells (specified during early embryonic development) assume a peripheral position in the larvae. In the Amphimedon parenchymella, this process occurs by non-polarized cell migration, resulting in formation of the outer layer composed of small, ciliated cells, excluded from the posterior pole [60] . In the Sycon amphiblastula, the small ciliated cells move as an epithelial sheet through an opening between the macromeres (in the process referred to as inversion, eversion or excurvation) [30] , [37] . In both cases, during metamorphosis, these ciliated cells then move to the inside, transdifferentiate into choanocytes and organize into the choanocyte chamber or a cluster of chambers. Finally, the osculum opens at the apical end, completing the process of metamorphosis. Thus, to support the hypothesis of germ layer homology, we expect expression of endomesoderm regulators in the ciliated micromeres of the embryos and larvae, followed by expression of these genes in the choanocytes. Previous analysis of gene expression during embryonic development of Amphimedon is consistent with this view: all of the key components of the canonical Wnt pathway are expressed throughout the outer layer of embryos and larvae [42] . Here we demonstrated that the key components of the canonical Wnt pathway ( FzdA and FzdD , DvlA , β catA ) are specifically expressed in the micromeres ( Fig. 10a ), or are expressed broadly including the micromeres ( Lrp5/6 , Tcf ) of Sycon embryos and larvae. At least one gene representing each component class is also expressed in choanocytes, and some in mesohyl cells of adults, suggesting they continue to specify these cell types during growth of the sponge ( Fig. 10f ). We have extended our analysis beyond the Wnt pathway and analyzed expression of additional genes implicated in endomesoderm formation of cnidarians [19] : Smad1/5 and Smad4 , Brachyury , Pl10 , Vasa , Nanos and Gli , as well as Gata , a component of the endomesoderm specification kernel in bilaterians [2] . Except for Nanos , all of these genes are predominantly expressed in the micromeres of the embryos/larvae and the choanocytes ( Fig. 10b–f ), supporting the notion of homology of the germ layers. Thus, while sponges contain only a limited number of direct orthologues of genes involved in body plan patterning in the eumetazoans, all of them are expressed in patterns supporting Haeckel’s view that body plans of sponges and cnidarians are homologous: choanoderm corresponds to the gastrodermis and osculum to the mouth of the polyp. Clearly, the described expression patterns of the developmental regulatory genes, while highly suggestive, do not prove homology of the body plans. Rather, they provide the necessary first step and a framework for studies aimed at determining the regulatory networks governing development of sponges. Once established, these networks can be further compared with developmental regulatory networks in other animals and provide insights into the molecular mechanisms underlying diversification of animal body plans. Samples Adult S. ciliatum specimens were collected from fjords located near Bergen, Norway, every few weeks during the vitellogenesis phase and then every few days as embryonic development started ( Table 1 ). As we expected differential expression of some of the studied genes across the body axis (see below), only mid-body fragments were used to investigate expression changes during oogenesis and embryonic development. Each individual sponge was dissected and part of it subjected to histological analysis to determine the developmental stage, and part used for total RNA isolation using the AllPrep DNA/RNA Mini Kit (Qiagen). Pools of samples derived from sponges containing the same developmental stages were used to generate Illumina RNA-Seq libraries, with biological replicates obtained wherever possible (Table1). We distinguish nine embryonic stages: early (small oocytes) and late vitellogenesis (medium to large oocytes, but no fertilization complex visible on histological analysis); fertilization (large oocytes, many of which are in fertilization complex as described [30] , [37] and shown in Fig. 1h ); early cleavage (2–16 cells); late cleavage (multiple cells, but no differentiation of cells apparent); early preinversion (cilia of micromeres visible); late preinversion (embryonic epithelium folding out in the centre); early postinversion (embryos in the choanocyte chamber, their cavities communicating with the mesohyl) and late postinversion (no connection between the embryonic cavity and the mesohyl; the embryos are free in the radial chambers and ready for release). We also isolated RNA from released larvae without the accompanying adult tissue: sponges containing larvae were kept in plastic cups until the larvae were released; larvae were either processed for RNA isolation, or placed in sterile filtered sea water in petri dishes for settlement. To gain insight into gene expression during maintenance of the adult body plan, we also constructed libraries from axially dissected non-reproductive specimens (that is, those in which we were unable to detect oocytes by histological analysis) collected in October, outside of the reproductive season. In this experiment, samples were collected in triplicates for top and bottom parts of the sponges, as well as two sets of adjacent middle samples (six middle samples in total; Table 1 ). Genomic DNA was isolated from non-reproductive single specimens and juveniles grown in the laboratory in semi-sterile conditions using the AllPrep DNA/RNA Mini Kit (Qiagen) as in case of RNA isolation. Sequencing Complementary DNA and genomic libraries were constructed and sequenced using Illumina technology at The Norwegian High-Throughput Sequencing Centre (all samples except juvenile-derived DNA) and DNA Facility Next Generation Sequencing Service at Iowa State University (juvenile-derived DNA). After de-novo assemblies of the genome and transcriptome, S. ciliatum genomic scaffolds and complementary DNA contigs were identified by aligning them with juvenile-derived (and therefore devoid of eukaryotic contaminations) genomic sequences. Phylogenetic analysis Phylogenetic gene trees were built using the MrBayes package (Bayesian inference) [61] modified to incorporate the LG substitution model. Model parameters were estimated using the ProtTest3 package [62] . MrBayes was set to run two sets of four Markov chains. The simulations were stopped once, at least 1 M iterations passed after split frequency between the two runs reached level lower than 0.01. Expression analysis Calculation and statistical analysis of the gene expression levels from the RNA-Seq data were performed using the RSEM [49] and the DESeq [50] packages. Expression level was calculated as sum of the posterior probability of each read coming from a given gene over all reads, the ‘expected_count’ from RSEM scaled (divided) by size factors of the RNA-Seq libraries calculated by DESeq. Calculation of statistical significance of gene expression being different (higher) in the apical part of the sponge was based on analysis of the negative binomial distribution of the expression levels [50] . We have used the DESeq ‘padj’, P -value adjusted for multiple testing with the Benjamini-Hochberg procedure with cutoff ≤0.1 for calling the expression significantly different. Reproducibility of the results was assessed by Principal Component Analysis and sample-to-sample distances [50] (see supplementary materials for details). In situ hybridization Approximately 1 kb long coding sequence probes were cloned and in situ hybridization was performed as described [34] , except for released larvae, which after fixation and washing in 70% ethanol were transferred to 100% ethanol and air dried on polyL-lysine-treated microscope cover slips before in situ hybridization and detection. Accession codes: DNA sequences generated in this study have been deposited at the European Nucleotide Archive under accession codes HG973349 to 973421 ( http://www.ebi.ac.uk/ena/data/view/HG973349-HG973421 ). RNA-seq data have been deposited in the ArrayExpress database, www.ebi.ac.uk/arrayexpress under accession codes E-MTAB-2430 and E-MTAB-2431 . How to cite this article: Leininger, S. et al. Developmental gene expression provides clues to relationships between sponge and eumetazoan body plans. Nat. Commun. 5:3905 doi: 10.1038/ncomms4905 (2014).